Inorganic hole conductor-based lead halide perovskite solar cells with 12.4% conversion efficiency Organo-lead halide perovskites have attracted much attention for solar cell applications due to their unique optical and electrical properties. With either low-temperature solution processing or vacuum evaporation, the overall conversion efficiencies of perovskite solar cells with organic hole-transporting material were quickly improved to over 15% during the last 2 years. However, the organic hole-transporting materials used are normally quite expensive due to complicated synthetic procedure or high-purity requirement. Here, we demonstrate the application of an effective and cheap inorganic p-type hole-transporting material, copper thiocyanate, on lead halide perovskite-based devices. With low-temperature solution-process deposition method, a power conversion efficiency of 12.4% was achieved under full sun illumination. This work represents a well-defined cell configuration with optimized perovskite morphology by two times of lead iodide deposition, and opens the door for integration of a class of abundant and inexpensive material for photovoltaic application. The hybrid organic–inorganic methylammonium lead halide perovskites (CH 3 NH 3 PbX 3 , X=Cl − , Br − , I − ) pioneered for use in thin-film transistors by Mitzi and colleagues [1] , and introduced as a light harvester in dye sensitized solar cell configurations by Miyasaka and colleagues [2] , have attracted intense attention for thin-film photovoltaics, due to their large absorption coefficient, high charge carrier mobility and diffusion length [3] , [4] , [5] , [6] , [7] , [8] , [9] , [10] , [11] , [12] , [13] , [14] , [15] . Power conversion efficiencies (PCEs) of over 15% were obtained with both mesoporous metal oxide scaffold and in planar heterojunction architectures [16] , [17] , [18] . Despite the rapid increase in efficiency associated with the evolution of different types of perovskites and device fabrication techniques, the HTM used were mainly limited to organic compounds, the state-of-the-art 2,2′,7,7′-tetrakis( N , N -di-p-methoxyphenylamine)-9,9′-spirobifluorene (spiro-MeOTAD) [16] , [17] , [18] and other small molecules, such as pyrene arylamine derivatives [19] and conducting polymers [20] , [21] , [22] . Their relatively high cost when compared with the n-type semiconductors (TiO 2 , ZnO) and to the perovskite itself is one of the main limitation of these materials for further large-scale application. Compared with organic HTMs, inorganic p-type semiconductors appear to be an ideal choice given their high mobility, stability, ease of synthesis and low cost. Copper iodide (CuI) was just reported as a hole conductor in lead halide perovskite-based devices, showing a PCE of 6% (ref. 23 ). Another interesting inorganic p-type semiconductor is copper thiocyanate (CuSCN), which shows good transparency throughout the visible and near infrared spectrum, high hole mobility of 0.01–0.1 cm 2 V −1 s −1 (as compared with 4 × 10 −5 cm 2 V −1 S −1 for spiro-MeOTAD) and good chemical stability [24] , [25] , [26] , [27] . Furthermore, it can be deposited through a solution-processed processing at low temperature, making it compatible with also flexible substrates. Herein, we demonstrate a device structure consisting of titanium dioxide as a scaffold as well as electron collector, lead halide perovskite as the light harvester and CuSCN as the HTM. The combination of CH 3 NH 3 PbI 3 perovskite with CuSCN shows high PCE of 12.4% under full sun illumination, indicating their further application in cost-effective photovoltaic devices. Device structure The solar cell configuration and the energy level diagram of the materials used are shown in Fig. 1 . The commercially available fluorine-doped tin oxide (FTO) glass substrate was first covered with a thin TiO 2 compact underlayer ( ∼ 50 nm) as hole-blocking layer before spin-coating a colloidal anatase paste to form a mesoporous TiO 2 film (electron extracting scaffold). The light harvester, CH 3 NH 3 PbI 3 , was then introduced using a sequential deposition method where the lead iodide (PbI 2 ) solution was spin-coated on the photoanode before dip-coating the TiO 2 /PbI 2 film into a CH 3 NH 3 I solution [16] . After annealing, the p-type HTM CuSCN was introduced by doctor-blading technique to ensure effective hole extraction and collection at the Au cathode. 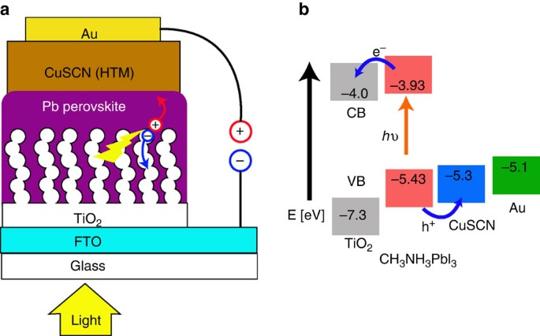Figure 1: Device architecture and energy level diagram. (a) Schematics cross-sectional view of the perovskite solar cell configuration: FTO glass, compact TiO2underlayer, mesoporous TiO2with infiltrated CH3NH3PbI3, CuSCN HTM, and gold. (b) Energy level diagram of the TiO2/CH3NH3PbI3/CuSCN/Au device showing ideal electron injection and hole extraction. Figure 1: Device architecture and energy level diagram. ( a ) Schematics cross-sectional view of the perovskite solar cell configuration: FTO glass, compact TiO 2 underlayer, mesoporous TiO 2 with infiltrated CH 3 NH 3 PbI 3 , CuSCN HTM, and gold. ( b ) Energy level diagram of the TiO 2 /CH 3 NH 3 PbI 3 /CuSCN/Au device showing ideal electron injection and hole extraction. 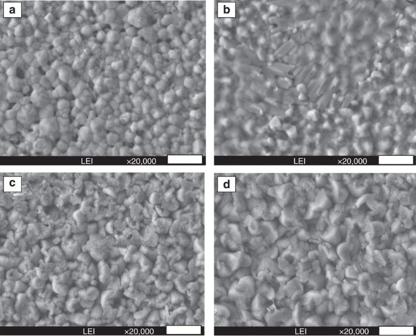Figure 2: Surface coating and structures by SEM. (a) TiO2/CH3NH3PbI3(single deposition). (b) TiO2/CH3NH3PbI3(double deposition). (c) TiO2/CH3NH3PbI3(single deposition)/CuSCN. (d) TiO2/CH3NH3PbI3(double deposition)/CuSCN. Scare bar, 1 μm. Full size image Figure 2 shows the top-surface scanning electron microscopy (SEM) images of the TiO 2 /CH 3 NH 3 PbI 3 electrodes without ( Fig. 2a,b ) and with ( Fig. 2c,d ) CuSCN. In order to maximize the light harvesting by CH 3 NH 3 PbI 3 layer, the loading of the mesoporous TiO 2 with PbI 2 was carried up from one time (1 × PbI 2 , single deposition) to two times (2 × PbI 2 , double deposition), followed by brief exposure to the methylammonium iodide solution in isopropanol as described elsewhere resulting in the conversion of PbI 2 to the perovskite CH 3 NH 3 PbI 3 (ref. 16 ). In both cases, the mesoporous TiO 2 was fully covered with a thin CH 3 NH 3 PbI 3 overlayer. However, when comparing top-surface images of the single versus double PbI 2 deposition, it is found that the perovskite overlayer is still porous in the first case but more uniform and dense when the PbI 2 is deposited twice. The addition of CuSCN can completely coat the CH 3 NH 3 PbI 3 , but the CuSCN crystal size formed from the single PbI 2 deposition film ( Fig. 2c ) is smaller. Therefore, the CuSCN lies close to the TiO 2 surface due to its filling into the remaining pores of the perovskite film. Thus, it is expected that the single PbI 2 depositon would not efficiently block contacts between the TiO 2 and HTM or the CH 3 NH 3 PbI 3 and Au. Figure 2: Surface coating and structures by SEM. ( a ) TiO 2 /CH 3 NH 3 PbI 3 (single deposition). ( b ) TiO 2 /CH 3 NH 3 PbI 3 (double deposition). ( c ) TiO 2 /CH 3 NH 3 PbI 3 (single deposition)/CuSCN. ( d ) TiO 2 /CH 3 NH 3 PbI 3 (double deposition)/CuSCN. Scare bar, 1 μm. 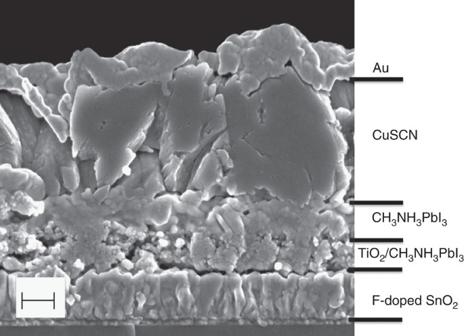Figure 3: Cross-section of the complete device by SEM. TiO2/CH3NH3PbI3(2 × PbI2, double deposition)/CuSCN/Au. Scale bar, 200 nm. Full size image Figure 3 shows a cross-sectional SEM picture of the complete device with the structure of FTO glass/TiO 2 /CH 3 NH 3 PbI 3 /CuSCN/Au. The overlayer of CH 3 NH 3 PbI 3 between TiO 2 /CH 3 NH 3 PbI 3 and CuSCN is ∼ 200 nm. The deposition of the CuSCN HTM by doctor blading forms a ∼ 600 nm capping layer, efficiently blocking contact between CH 3 NH 3 PbI 3 and Au. Figure 3: Cross-section of the complete device by SEM. TiO 2 /CH 3 NH 3 PbI 3 (2 × PbI 2 , double deposition)/CuSCN/Au. Scale bar, 200 nm. Full size image In order to qualitatively study the effect of PbI 2 deposition on CH 3 NH 3 PbI 3 loading, SEM-electron probe microanalyser (EPMA) elemental analysis on the samples cross section have been performed. Elemental mapping by SEM is helpful in examining the quantitative composition and distribution of constituents throughout the device. The elemental mappings of titanium, lead, copper and gold are shown in Fig. 4 . Please note that the small amount of Pb and Cu elements observed (blue pixels) above the Au cathode is due to eluted Pb and Cu cations from the CH 3 NH 3 PbI 3 and CuSCN during the cross-section preparation with focused ion beam. Indeed, minute amounts of pulverized metal ions are hard to avoid completely during ion bombardment and represent concentrations much lower that observed in high-concentration zone. Without CuSCN, the CH 3 NH 3 PbI 3 overlayer appears to be more uniform and non-porous with double deposition (2 × PbI 2 ) method ( Fig. 4b ). The concentration of Pb is also found to be significantly higher than that formed with single deposition (1 × PbI 2 ; Fig. 4a ). With the presence of CuSCN, Pb signal is observed above that of Ti, which would be expected for partial dissolution of the Pb perovskite overlayer during CuSCN deposition. Indeed, the splitting between regions of highest signal for Pb and Ti with double deposition was even larger ( Fig. 4d ), which is consistent with the dissolution of CH 3 NH 3 PbI 3 into CuSCN. As this dissolution effect might reduce the shunt resistance, proper capping of TiO 2 surface by CH 3 NH 3 PbI 3 is important for reducing the shunt between TiO 2 and CuSCN. A thick CH 3 NH 3 PbI 3 capping layer ( ∼ 200 nm) on the top of TiO 2 was obtained by double deposition, whereas with single deposition the capping layer might be too thin to properly isolate TiO 2 and CuSCN electrically. 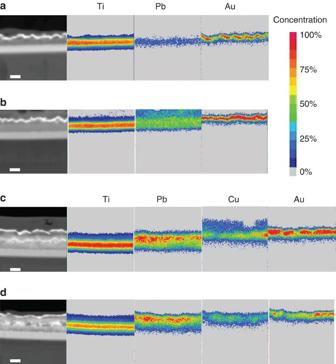Figure 4: Elemental analysis by SEM-EPMA. (a) TiO2/CH3NH3PbI3(single deposition)/Au. (b) TiO2/CH3NH3PbI3(double deposition)/Au. (c) TiO2/CH3NH3PbI3(single deposition)/CuSCN/Au. (d) TiO2/CH3NH3PbI3(double deposition)/CuSCN/Au. The upper bright line observed on the upper part of each cross-sectional s.e.m. is due to the Au cathode. Scare bar, 500 nm. Figure 4: Elemental analysis by SEM-EPMA. ( a ) TiO 2 /CH 3 NH 3 PbI 3 (single deposition)/Au. ( b ) TiO 2 /CH 3 NH 3 PbI 3 (double deposition)/Au. ( c ) TiO 2 /CH 3 NH 3 PbI 3 (single deposition)/CuSCN/Au. ( d ) TiO 2 /CH 3 NH 3 PbI 3 (double deposition)/CuSCN/Au. The upper bright line observed on the upper part of each cross-sectional s.e.m. is due to the Au cathode. Scare bar, 500 nm. 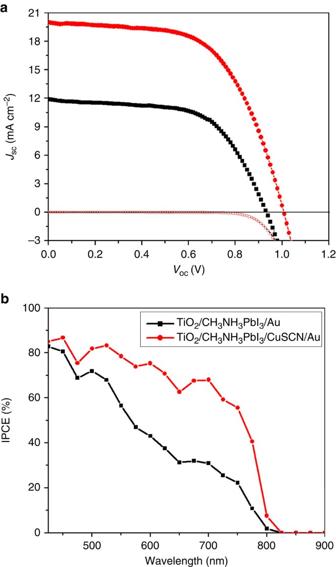Figure 5:J-Vand IPCE spectra. (a) Current–voltage characteristics of the heterojunction solar cells with (red) and without (black) CuSCN measured in the dark and under 100 mW cm−2photon flux (AM1.5G). (b) The corresponding IPCE spectra showing improved photocurrent with the addition of the CuSCN HTM. Full size image Photovoltaic performance Figure 5 showed the current–voltage ( J-V ) characteristics measured under dark and simulated AM1.5G (100 mW cm −2 ) irradiation for the champion device comprised of FTO/compact TiO 2 /mesoporous TiO 2 /CH 3 NH 3 PbI 3 (double deposition)/CuSCN/Au. A reference cell without HTM was fabricated under the same conditions for comparison. The device with CuSCN displayed a short circuit current density ( J sc ) of 19.7 mA cm −2 , an open-circuit voltage ( V oc ) of 1,016 mV and a fill factor ( FF ) of 0.62, leading to a PCE of 12.4%. Without CuSCN, the device shows a PCE of 6.7%, with a significant decrease in both the J sc (from 19.7 mA cm −2 to 11.9 mA cm −2 ) and V oc (from 1,016 mV to 933 mV). Table 1 shows the photovoltaic parameters of the best cells and the average of a selection of cells made under the same conditions. The high J sc obtained with CuSCN is mainly due to the effective charge extraction between CH 3 NH 3 PbI 3 and CuSCN, followed by fast hole transport through CuSCN to the Au. Here, the high hole mobility in CuSCN enabled high J sc in the cell with the optimized 600–700 nm thick HTM overlayer. Further improvement of the thickness of CuSCN overlayer gave compatible conversion efficiencies. When comparing the incident photon-to-current conversion efficiency (IPCE) spectra for cells with and without CuSCN ( Fig. 5b ), the presence of CuSCN is found to enable significantly higher internal quantum efficiency contributing to a higher photocurrent between 450 nm to 800 nm and further confirm efficient charge injection and collection. Indeed, the IPCE spectrum shows a sharp rise at 800 nm to reach 55% at 750 nm and close to 85% IPCE at 400 nm. We also found a significant increase in V oc when using CuSCN as HTM to reach more than 1 V. Figure 5: J - V and IPCE spectra. ( a ) Current–voltage characteristics of the heterojunction solar cells with (red) and without (black) CuSCN measured in the dark and under 100 mW cm −2 photon flux (AM1.5G). ( b ) The corresponding IPCE spectra showing improved photocurrent with the addition of the CuSCN HTM. Full size image Table 1 Photovoltaic parameters derived from J - V measurements of CH 3 NH 3 PbI 3 -based devices with and without CuSCN HTM. Full size table The photovoltaic parameters of the single and double deposition of PbI 2 are shown in Table 1 . With the presence of CuSCN, the differences of J sc and V oc were negligible between single and double deposition, mainly the FF was improved. From the fitting of the I – V curves, the series and shunt resistances for single deposition were calculated to be 12.6 Ω·cm 2 and 956 Ω·cm 2 , respectively, which were changed to be 11.3 Ω·cm 2 and 3,580 Ω·cm 2 for double deposition. Such significant difference in shunt resistance can explain the improvement of FF from 0.56 to 0.62, and also the improved PCE. The V oc for the device without CH 3 NH 3 PbI 3 (TiO 2 /CuSCN/Au) was only 345 mV, which was 671 mV lower than that of our champion cell. Therefore, if there is a direct contact between TiO 2 and CuSCN, the accumulated charge can effectively pass through the contact and recombine. If the CH 3 NH 3 PbI 3 was indeed being partly redissolved when depositing the CuSCN, it would lead to an increased contact between TiO 2 and CuSCN. Therefore, a thick perovskite overlayer was necessary to avoid the unfavourable charge recombination. In our experiments, a higher shunt resistance was observed with double deposition method and resulted in an improved FF and PCE. In summary, we have demonstrated the application of an effective inorganic p-type HTM, CuSCN, by solution-process deposition on CH 3 NH 3 PbI 3 -based solar cells. The presence of CuSCN leads to an improvement in the overall efficiency to 12.4% through a 65% increase in short circuit current and 9% in open-circuit potential when comparing with the device without HTM. The high short circuit current and IPCE values indicate efficient charge extraction and collection from the excited CH 3 NH 3 PbI 3 to TiO 2 and CuSCN, respectively, and then to the corresponding electrodes. The EPMA mapping reveals a well-defined cell configuration hinting at partial dissolution of the perovskite by CuSCN. Consisting with this, the thicker perovkiste overlayer obtained with double PbI 2 deposition method shows to be superior with a higher shunt resistance and photovoltaic performance. Even with significant price variations with market size, comparing with typical organic HTMs (most often >> 100 USD per gram), CuSCN ( ∼ 1 USD per gram) shows almost two orders of magnitude lower price, making it more promising for large-scale application. This study opens the door for integration of a new class of abundant and inexpensive inorganic HTM for further printable photovoltaics application, and carbon neutral electricity production. Solar cell fabrication The F-doped SnO 2 coated glass substrate (FTO, TEC-15 ( t =2 mm), NSG-Pilkington) was cleaned with detergent, water and ethanol, respectively, and then treated with a ultraviolet/O 3 cleaner for 15 min. The compact TiO 2 layer was coated on FTO substrate by spray pyrolysis using a precursor solution of titanium di-isopropoxide bis(acetylacetonate; 0.6 ml titanium acetylacetonate in 8 ml ethanol) on a hot plate at 500 °C. The titanium acetylacetonate was prepared by pouring acetylacetone (Wako Pure Chemical Industries, Ltd.) into titanium isopropoxide (Kanto Chemical Co., Inc.) with a mole ratio of 2:1. For the preparation of mesoporous TiO 2 layer, a commercial TiO 2 paste (2 g, 20 nm particle size, PST-18NR, JGC Catalysts and Chemicals Ltd., Japan) was diluted with ethanol (7 g), and spin-coated on the prepared substrate at 5,000 r.p.m. for 25 s (5 s acceleration). After drying at 125 °C, the film was annealed at 500 °C in air. PbI 2 was dissolved in N,N -dimethylformamide to yield a 1.3 M solution under stirring at 70 °C. The PbI 2 solution (50 μl) was deposited on the mesoporous TiO 2 film by spin-coating at 6,500 r.p.m. for 18 s (2 s acceleration), followed by drying at 70 °C for 30 min. For each PbI 2 deposition, the mesoporous TiO 2 films were heated using a hot plate at 70 °C. After that, the prepared TiO 2 /PbI 2 film was dipped in a solution of CH 3 NH 3 I in 2-propanol (10 mg ml −1 ) for 20 s, rinsed with 2-propanol and and dried at 70 °C for 30 min. The CuSCN HTM was then deposited by doctor blading at 65 °C. The solution was prepared by dissolving 6 mg CuSCN (Kishida Chemical Co. Ltd.) in 1 ml propyl sulfide. Finally, 50 nm of gold was evaporated on top as the back contact. Photovoltaic characterization Current–voltage characteristics were recorded by applying an external potential bias to the cell and recording the generated photocurrent with a digital source metre (6240, ADCMT). The light source was a 500 W xenon lamp equipped with a sunlight filter (YSS-100A, Yamashita Denso Co. Ltd.) to match the emission spectrum of the lamp to the AM1.5G standard. Before each measurement, the light intensity was calibrated with a silicon reference cell. For the I – V measurement, the voltage step and delay time were 10 mV and 1 ms, respectively. The scan started from 0 V (the short circuit condition) to 1.1 V (over the open-circuit photovoltage). IPCE measurements were determined using a 300 W xenon light source and a monochromator. The devices were masked with a black metal aperture to define the active area of 0.09 cm 2 . SEM The top-surface and cross-sectional images were investigated using a high-resolution scanning electron microscope (JEOL JSM-7400F, accelerating voltage: 15 kV). Images were obtained with an in-lens secondary electron detector. EPMA for Elemental Analysis were done by using JEOL JXA-8500F. The accelerating voltage for the EPMA–wavelength dispersive spectroscopy measurements was 10 kV. In order to improve the spatial resolution, each sample was fixed in the glue and sliced out by focused ion beam to avoid enlarged interaction volume passed through the observing surface. How to cite this article: Qin, P. et al. Inorganic hole conductor-based lead halide perovskite solar cells with 12.4% conversion efficiency. Nat. Commun. 5:3834 doi: 10.1038/ncomms4834 (2014).